GRK6 deficiency in mice causes autoimmune disease due to impaired apoptotic cell clearance Efficient engulfment of apoptotic cells is critical for maintaining tissue homoeostasis. When phagocytes recognize ‘eat me’ signals presented on the surface of apoptotic cells, this subsequently induces cytoskeletal rearrangement of phagocytes for the engulfment through Rac1 activation. However, the intracellular signalling cascades that result in Rac1 activation remain largely unknown. Here we show that G-protein-coupled receptor kinase 6 (GRK6) is involved in apoptotic cell clearance. GRK6 cooperates with GIT1 to activate Rac1, which promotes apoptotic engulfment independently from the two known DOCK180/ELMO/Rac1 and GULP1/Rac1 engulfment pathways. As a consequence, GRK6-deficient mice develop an autoimmune disease. GRK6-deficient mice also have increased iron stores in splenic red pulp in which F4/80 + macrophages are responsible for senescent red blood cell clearance. Our results reveal previously unrecognized roles for GRK6 in regulating apoptotic engulfment and its fundamental importance in immune and iron homoeostasis. During animal development and in immune responses, numerous harmful and unnecessary cells are generated. These cells undergo apoptosis and are rapidly engulfed by phagocytes such as macrophages and dendritic cells. When an engulfment system does not function adequately, dying cells accumulate and undergo secondary necrosis that results in the release of noxious cellular components into the extracellular space. These released self-antigens are considered to induce lymphocyte activation and autoantibody production, which results in the development of autoimmune diseases such as systemic lupus erythematosus (SLE). Thus, the efficient clearance of apoptotic cells is indispensable for maintaining tissue homoeostasis. Apoptotic cell removal is supposedly triggered by the release of ‘find me’ signals such as nucleotides and lipids from dying cells [1] . These signals recruit phagocytes to the apoptotic cells. Subsequently, the recruited phagocytes recognize ‘eat me’ signals on the surface of apoptotic cells through the corresponding phagocyte receptors [2] . This receptor recognition then elicits signals that induce cytoskeletal rearrangements for encapsulating the apoptotic cells [3] . To date, a variety of ligands on apoptotic cells and their corresponding receptors on phagocytes have been proposed to be involved in this recognition process [4] . Two conserved intracellular pathways, CrkII/DOCK180/ELMO/Rac1 and GULP/Rac1, are well known to be involved in cytoskeletal rearrangements for apoptotic cell engulfment [5] , [6] , [7] . However, molecules downstream of phagocytic receptors that are required for ingesting apoptotic cells still remain much to be determined. G-protein-coupled receptor kinase 6 (GRK6) is a member of the GRK superfamily. GRKs were initially identified as molecules that phosphorylate G-protein-coupled receptors (GPCRs) and result in their desensitization [8] , [9] , [10] . When GPCRs are activated by binding to their cognate ligands, GRKs recognize these activated receptors and phosphorylate them. Then, β-arrestins bind to these phosphorylated receptors, which block further stimulation of G-proteins by the agonist-bound receptors through steric hindrance [11] . In addition to regulating GPCR desensitization, recent evidence indicates that GRKs have roles in cellular signalling independently of the GPCR-mediated pathways by phosphorylating non-GPCR substrates [12] , [13] . For example, GRK2 and GRK5 phosphorylate IRS1 and HDAC5, respectively [14] , [15] . Although numerous in vitro studies have established the importance of GRKs for regulating GPCR signalling and phosphorylating non-GPCR proteins, the physiological and pathological roles of GRKs, including GRK6, in vivo remain poorly understood. Here we demonstrate a previously unknown function for GRK6 in apoptotic cell clearance. GRK6 enhances apoptotic cell engulfment through Rac1 activation, an indispensable molecule involved in engulfment signalling. In addition, we show that this GRK6-mediated engulfment depends on GIT1 [16] and phosphorylation of radixin and moesin [17] , both of which have been implicated in membrane skeleton organization. GRK6-deficient macrophages exhibited impaired phagocytosis of apoptotic cells. Consequently, GRK6-deficient mice developed an autoimmune condition similar to those of mice with other knocked-out molecules involved in apoptotic engulfment. We also found that GRK6 was highly expressed in red splenic macrophages responsible for removing senescent red blood cells. GRK6 significantly contributed to their clearance, as GRK6-deficient mice had increased iron stores because of the inefficient iron uptake in the red pulp of their spleens. Our results establish that GRK6 is a critical factor for regulating immune and iron homoeostasis. GRK6 is involved in the engulfment of apoptotic cells To examine the possible involvement of GRK family members in the engulfment of apoptotic cells, we first examined the effects of GRKs on the engulfment by NIH3T3 cells. NIH3T3 is a mouse embryonic fibroblast cell line, although these cells can engulf apoptotic thymocytes. In addition, the efficiency of retroviral gene transfer to these cells is >90%. Thus, we used NIH3T3 cells as phagocytes in our experiments. Among the seven GRKs, some GRK (GRK1, 4 and 7) expressions are restricted to certain tissues, whereas other GRKs (GRK2, 3, 5 and 6) are widely expressed [18] . Thus, we introduced kinase-inactive and dominant-negative (DN) mutants [19] of GRK2, 3, 5 and 6 (GRK2 (K220R), GRK3 (K220R), GRK5 (K215R) and GRK6 (K215R)) into NIH3T3 cells and determined the effect of each mutant on NIH3T3 cells’ engulfment capacity. Virally infected NIH3T3 cells were co-cultured with fluorescently labelled apoptotic thymocytes at 37 °C for 90 min. After co-culture, the fluorescence uptake by NIH3T3 cells was evaluated by flow cytometry. As shown in Fig. 1a , 18% of the vector-expressing NIH3T3 cells engulfed apoptotic cells under these experimental conditions. Among the four kinase-inactive and DN GRK mutants, only GRK6 (K215R) significantly attenuated apoptotic cell engulfment by NIH3T3 cells, which indicated that GRK6 kinase activity was important for efficient engulfment ( Fig. 1a ). Knockdown of GRK6 by small interfering RNA (siRNA) treatment (about 70% reductions in the GRK6 protein level) also reduced the engulfment by NIH3T3 cells ( Fig. 1b ). Conversely, overexpression of GRK6 increased engulfment by NIH3T3 cells ( Fig. 1c ). These results demonstrated that GRK6 enhanced the clearance of apoptotic cells. In contrast to GRK6, GRK2 (K220R) expression increased apoptotic engulfment ( Fig. 1a ). However, GRK2 knockdown by siRNA resulted in significantly decreased engulfment, and overexpression of GRK2 greatly increased engulfment ( Supplementary Fig. S1 ). These results indicated that GRK2 could enhance engulfment independent of its kinase activity, which is similar to the role of GRK2 in cell migration [20] . 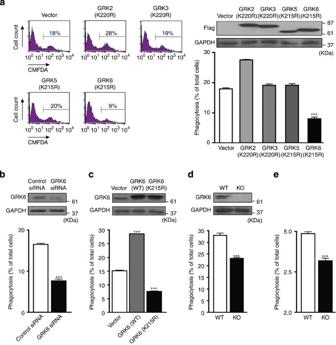Figure 1: Involvement of GRK6 in the engulfment of apoptotic cells. (a) NIH3T3 cells were infected with the empty retrovirus vector or the virus carrying the cDNA for kinase-inactive form of GRK2, GRK3, GRK5 or GRK6 (GRK2 (K220R), GRK3 (K220R), GRK5 (K215R) or GRK6 (K215R)) with N-terminal Flag tag. The infected cells (4 × 104cells) were co-cultured with CMFDA-labelled WT thymocytes (1 × 106cells) at 37 °C for 90 min. Percentages of the phagocytes carrying the engulfed thymocytes were determined by FACS as detailed in Methods. The representative FACS profiles with the NIH3T3 cells expressing GRK2 (K220R), GRK3 (K220R), GRK5 (K215R) or GRK6 (K215R) are shown from four independent experiments performed in triplicate. The expression level of each GRK mutant in NIH3T3 cells was determined by immunoblot analysis using anti-Flag and anti-GAPDH antibodies. (b) The engulfment ability of NIH3T3 cells transfected with control or GRK6 siRNA was estimated by FACS analysis as described ina. The cell lysates of the NIH3T3 cells were analysed by western blot with antibody against GRK6 or GAPDH. Expression level of GRK6 was decreased to about 30% of the normal level following treatment with GRK6 siRNA. (c) The engulfment ability of NIH3T3 cells expressing GRK6 (WT) or GRK6 (K215R) was evaluated by FACS as described ina. The level of GRK6 (WT) or GRK6 (K215R) was more than 10-fold greater than endogenous levels, determined by immunoblot using anti-GRK6 antibody. (d) BMDMs (1 × 105cells) from WT and GRK6-deficient mice were co-cultured with CMFDA-labelled apoptotic thymocytes (1 × 106cells) at 37 °C for 60 min. The percentage of the phagocytes carrying the engulfed thymocytes is presented. BMDM lysates from WT and GRK6-deficient mice were analysed by western blot with antibody against GRK6 or GAPDH. (e) CMFDA-labelled apoptotic thymocytes (8 × 107cells) were injected to WT and GRK6-deficient mice from tail vein. Two hours after the injection, their spleens were isolated and stained with anti-CD11b antibody. Percentage of CD11b+splenic macrophage carrying the labelled thymocytes was evaluated by flow cytometer. All the experiments were done at least three times; all graphs show average with s.e.m. ***P<0.001. KO, knockout. Figure 1: Involvement of GRK6 in the engulfment of apoptotic cells. ( a ) NIH3T3 cells were infected with the empty retrovirus vector or the virus carrying the cDNA for kinase-inactive form of GRK2, GRK3, GRK5 or GRK6 (GRK2 (K220R), GRK3 (K220R), GRK5 (K215R) or GRK6 (K215R)) with N-terminal Flag tag. The infected cells (4 × 10 4 cells) were co-cultured with CMFDA-labelled WT thymocytes (1 × 10 6 cells) at 37 °C for 90 min. Percentages of the phagocytes carrying the engulfed thymocytes were determined by FACS as detailed in Methods. The representative FACS profiles with the NIH3T3 cells expressing GRK2 (K220R), GRK3 (K220R), GRK5 (K215R) or GRK6 (K215R) are shown from four independent experiments performed in triplicate. The expression level of each GRK mutant in NIH3T3 cells was determined by immunoblot analysis using anti-Flag and anti-GAPDH antibodies. ( b ) The engulfment ability of NIH3T3 cells transfected with control or GRK6 siRNA was estimated by FACS analysis as described in a . The cell lysates of the NIH3T3 cells were analysed by western blot with antibody against GRK6 or GAPDH. Expression level of GRK6 was decreased to about 30% of the normal level following treatment with GRK6 siRNA. ( c ) The engulfment ability of NIH3T3 cells expressing GRK6 (WT) or GRK6 (K215R) was evaluated by FACS as described in a . The level of GRK6 (WT) or GRK6 (K215R) was more than 10-fold greater than endogenous levels, determined by immunoblot using anti-GRK6 antibody. ( d ) BMDMs (1 × 10 5 cells) from WT and GRK6-deficient mice were co-cultured with CMFDA-labelled apoptotic thymocytes (1 × 10 6 cells) at 37 °C for 60 min. The percentage of the phagocytes carrying the engulfed thymocytes is presented. BMDM lysates from WT and GRK6-deficient mice were analysed by western blot with antibody against GRK6 or GAPDH. ( e ) CMFDA-labelled apoptotic thymocytes (8 × 10 7 cells) were injected to WT and GRK6-deficient mice from tail vein. Two hours after the injection, their spleens were isolated and stained with anti-CD11b antibody. Percentage of CD11b + splenic macrophage carrying the labelled thymocytes was evaluated by flow cytometer. All the experiments were done at least three times; all graphs show average with s.e.m. *** P <0.001. KO, knockout. Full size image Next, we examined if GRK6 mediated apoptotic cell engulfment by macrophages. Bone marrow-derived macrophages (BMDMs) from wild-type (WT) mice expressed GRK6 ( Supplementary Fig. S2 ) and efficiently engulfed apoptotic thymocytes. In comparison, BMDMs from GRK6-deficient mice had a significantly decreased ability to engulf apoptotic cells ( Fig. 1d ). GRK6-deficient BMDMs also had decreased uptake of fluorescent microspheres, although the extent of this decrease was less than that observed for apoptotic cell engulfment ( Supplementary Fig. S3 ). We further examined the contribution of GRK6 to apoptotic cell clearance by macrophages in vivo . Fluorescently labelled apoptotic thymocytes were injected into WT and GRK6-deficient mice. Phagocytosis by splenic macrophages from GRK6-deficient mice was approximately one-third less than that by macrophages from WT mice, which indicated that engulfment was impaired in GRK6-deficient splenic macrophages ( Fig. 1e ). Collectively, GRK6 contributes to the efficient engulfment of apoptotic cells in various types of phagocytes, including macrophages. GRK6 operates upstream of Rac1 for engulfment To determine the molecular mechanisms by which GRK6 enhances apoptotic engulfment, we examined whether Rac1 participated in the GRK6-mediated engulfment pathway. Rac1 is an indispensable molecule for apoptotic cell engulfment [3] . Consistent with the results of a previous study [21] , a DN Rac1 mutant, Rac1 (T17N), almost completely inhibited engulfment by NIH3T3 cells. WT Rac1 expression markedly enhanced engulfment, which confirmed Rac1’s indispensable role in engulfment ( Fig. 2a ). Next, we co-expressed WT GRK6 and DN Rac1, Rac1 (T17N). Rac1 (T17N) expression completely abolished the enhanced engulfment induced by GRK6 ( Fig. 2a ). In contrast, GRK6 (K215R) expression did not significantly affect Rac1-promoted engulfment ( Fig. 2b ). The formation of lamellipodia that is characteristic for Rac1 activation [22] was observed in GRK6-expressing cells, whereas GRK6 (K215R) and Rac1 (T17N) expression significantly attenuated the formation of lamellipodia ( Supplementary Fig. S4 ). These morphological results together with our other data regarding engulfment suggested that GRK6 activated Rac1. We next examined the effect of GRK6 on Rac1 activity using a pull-down assay with the Rac1-binding domain of PAK (PAK-RBD), which specifically binds to the GTP form of Rac1. As shown in Fig. 2c , this pull-down assay showed that GRK6 overexpression significantly increased the level of Rac1-GTP, whereas the expression of GRK6 (K215R) decreased it. These results indicated that GRK6 enhanced engulfment through Rac1 activation. 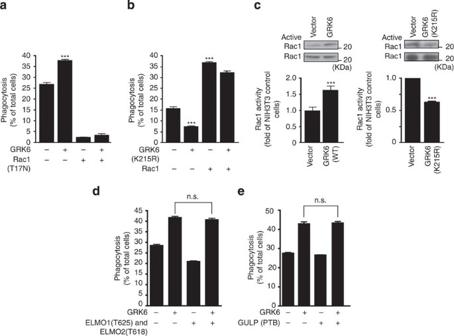Figure 2: GRK6 regulates engulfment of apoptotic cells via Rac1. (a,b) NIH3T3 cells were infected with retroviruses encoding WT GRK6 and DN Rac1 (T17N) (a), or kinase-inactive GRK6 (K215R) and WT Rac1 (b), either alone or in combination. The infected cells were subjected to the engulfment assay with CMFDA-labelled WT thymocytes. Percentages of the phagocytes carrying the engulfed thymocytes were determined by FACS. (c) NIH3T3 cells infected with the empty retrovirus vector or the virus carrying the cDNA for WT GRK6 were subjected to GTP-Rac1 pull-down assay using GST-CRIB. The pull-down samples were subjected to western blot using anti-Rac1 antibody and the level of GTP-bound Rac1 was quantified by densitometry, normalized against the total amount of Rac1 in the cell lysates. Data represent means±s.e.m. (error bars),n=3. (left panel) (d,e) NIH3T3 cells were infected with retroviral combinations of WT GRK6 and two DN forms of ELMO, ELMO1 (T625) and ELMO2 (T615) (d), retroviral combinations of WT GRK6 and a DN form of GULP, GULP (PTB), as indicated (e). The retrovirus-infected NIH3T3 cells were subjected to the engulfment assay. Percentages of the phagocytes carrying the engulfed thymocytes were determined by FACS. All the phagocytosis experiments were done at least three times, and the average numbers are shown with s.e.m. n.s., not significant. ***P<0.001. Figure 2: GRK6 regulates engulfment of apoptotic cells via Rac1. ( a , b ) NIH3T3 cells were infected with retroviruses encoding WT GRK6 and DN Rac1 (T17N) ( a ), or kinase-inactive GRK6 (K215R) and WT Rac1 ( b ), either alone or in combination. The infected cells were subjected to the engulfment assay with CMFDA-labelled WT thymocytes. Percentages of the phagocytes carrying the engulfed thymocytes were determined by FACS. ( c ) NIH3T3 cells infected with the empty retrovirus vector or the virus carrying the cDNA for WT GRK6 were subjected to GTP-Rac1 pull-down assay using GST-CRIB. The pull-down samples were subjected to western blot using anti-Rac1 antibody and the level of GTP-bound Rac1 was quantified by densitometry, normalized against the total amount of Rac1 in the cell lysates. Data represent means±s.e.m. (error bars), n =3. (left panel) ( d , e ) NIH3T3 cells were infected with retroviral combinations of WT GRK6 and two DN forms of ELMO, ELMO1 (T625) and ELMO2 (T615) ( d ), retroviral combinations of WT GRK6 and a DN form of GULP, GULP (PTB), as indicated ( e ). The retrovirus-infected NIH3T3 cells were subjected to the engulfment assay. Percentages of the phagocytes carrying the engulfed thymocytes were determined by FACS. All the phagocytosis experiments were done at least three times, and the average numbers are shown with s.e.m. n.s., not significant. *** P <0.001. Full size image GRK6 is part of a novel engulfment pathway The best-known and best-established intracellular molecular pathways involved in engulfment are the DOCK180/ELMO/Rac1 and GULP/Rac1 pathways, which have been identified in Caenorhabditis elegans and are conserved in mammals. These pathways supposedly operate in parallel, although in a partially redundant manner [5] . Thus, we examined if the GRK6-mediated engulfment pathway was related to these two signalling pathways. We generated DN ELMO mutants, ELMO1 and ELMO2, by truncating their C-terminal regions [23] and a DN GULP mutant by eliminating the phosphotyrosine-binding domain of GULP [24] and co-transfected these with GRK6. The expressions of both the ELMO mutants ( Fig. 2d ) and the GULP mutant ( Fig. 2e ) did not affect GRK6-mediated enhancement of apoptotic cell engulfment. These results suggested that the GRK6-mediated engulfment pathway was largely independent of two known pathways. GIT1 enhances GRK6-mediated engulfment To search for molecules that could be involved in GRK6-mediated Rac1 activation, we focused on the GRK-interacting ADP ribosylation factor GTPase-activating protein1 (GIT1). GIT1 is one of the few non-receptor proteins that interact with GRK6 [25] . However, a functional relationship between GRK6 and GIT1 and the binding region of GIT1 required for this interaction have not been established. GIT1 is expressed in various types of tissues and cells [16] . We confirmed that GIT1 was expressed in NIH3T3 cells, BMDMs and splenic macrophages ( Supplementary Fig. S5a ). Furthermore, GRK6 deficiency did not affect GIT1 expression in BMDMs ( Supplementary Fig. S5b ). GIT1 expression alone slightly increased the engulfment of apoptotic cells by NIH3T3 cells ( Fig. 3a ). However, when GIT1 was co-expressed with GRK6, GIT1 enhanced GRK6-mediated engulfment ( Fig. 3a ). To identify the amino-acid residues or region of GIT1 that were responsible for GRK6-mediated engulfment, we made some point [26] and deletion [27] mutants of GIT1, as shown in Fig. 3b and Supplementary Fig. S6a . GIT1 (R39K) expression, which lacks the ADP ribosylation factor–GTPase-activator protein activity, had no effect on the GRK6-mediated engulfment ( Supplementary Fig. S6b ). In comparison, mutants that lacked the coiled-coil domain of GIT1, GIT1(ΔC) and GIT1(ΔAC) significantly attenuated the GRK6-mediated engulfment ( Fig. 3a ). These GIT1 mutants also inhibited the Rac1 activation by GRK6 ( Fig. 3c ). Immunoprecipitation experiments revealed that GRK6 interacted with GIT1 ( Fig. 3d ) independently of its kinase activity ( Fig. 3f ), although GRK6 directly phosphorylated GIT1 ( Supplementary Fig. S7 ). Because the coiled-coil domain-deleted GIT1 mutants did not immunoprecipitate with GRK6, the coiled-coil domain was important for its interaction with GRK6 ( Fig. 3d ). This GRK6/GIT1 complex did not affect the GIT1-regulated signalling pathways that were previously reported [20] ( Supplementary Fig. S8 ). 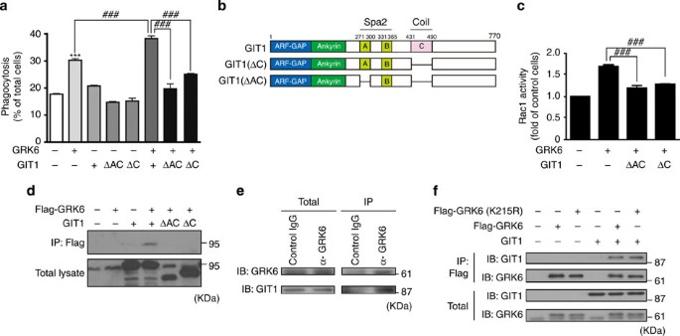Figure 3: GIT1 is involved in GRK6-mediated apoptotic engulfment. (a) NIH3T3 cells (4 × 104cells) infected with the indicated retroviruses were co-cultured at 37 °C for 90 min with 1 × 106cells CMFDA-labelled WT thymocytes. Percentages of the phagocytes carrying the engulfed thymocytes were determined by FACS. The experiments were done at least three times, and the average numbers are shown with s.e.m. (b) Schematic representation of GIT1 and its deletion mutants, GIT1 (ΔC) and GIT1 (ΔAC), used in this study. The numbers indicate the positions of the amino acids. (c) The activation state of Rac1 in NIH3T3 cells infected with the indicated retroviruses was measured in GTP-Rac1 pull-down assays with GST-CRIB. Data represent means±s.e.m. (error bars) of four independent experiments. (d) HEK293 cell lysates transiently transfected with the indicated plasmids were immunoprecipitated with anti-Flag antibody. Western blot was performed with anti-GIT1 antibody. (e) Cell extracts of BMDM from WT mice were immunoprecipitated with normal rabbit IgG or anti-GRK6 antibody. The total lysates and immunoprecipitates (IPs) of BMDMs were immunoblotted (IB) with anti-GRK6 and anti-GIT1 antibodies. (f) NIH3T3 cell lysates infected with the indicated retroviruses were immunoprecipitated with anti-Flag antibody. The IPs were subjected to western blot analysis with anti-GRK6 and anti-GIT1 antibodies. All the immunoprecipitation experiments were done at least three times, and representative data are shown. ***P<0.001,###P<0.001. Figure 3: GIT1 is involved in GRK6-mediated apoptotic engulfment. ( a ) NIH3T3 cells (4 × 10 4 cells) infected with the indicated retroviruses were co-cultured at 37 °C for 90 min with 1 × 10 6 cells CMFDA-labelled WT thymocytes. Percentages of the phagocytes carrying the engulfed thymocytes were determined by FACS. The experiments were done at least three times, and the average numbers are shown with s.e.m. ( b ) Schematic representation of GIT1 and its deletion mutants, GIT1 (ΔC) and GIT1 (ΔAC), used in this study. The numbers indicate the positions of the amino acids. ( c ) The activation state of Rac1 in NIH3T3 cells infected with the indicated retroviruses was measured in GTP-Rac1 pull-down assays with GST-CRIB. Data represent means±s.e.m. (error bars) of four independent experiments. ( d ) HEK293 cell lysates transiently transfected with the indicated plasmids were immunoprecipitated with anti-Flag antibody. Western blot was performed with anti-GIT1 antibody. ( e ) Cell extracts of BMDM from WT mice were immunoprecipitated with normal rabbit IgG or anti-GRK6 antibody. The total lysates and immunoprecipitates (IPs) of BMDMs were immunoblotted (IB) with anti-GRK6 and anti-GIT1 antibodies. ( f ) NIH3T3 cell lysates infected with the indicated retroviruses were immunoprecipitated with anti-Flag antibody. The IPs were subjected to western blot analysis with anti-GRK6 and anti-GIT1 antibodies. All the immunoprecipitation experiments were done at least three times, and representative data are shown. *** P <0.001, ### P <0.001. Full size image Radixin and moesin contribute to GRK6-mediated signalling To further characterize the GRK6-mediated pathway for apoptotic engulfment, we employed a newly developed phosphoproteomic approach to identify target proteins for GRK6 [28] . We prepared three phosphoprotein-enriched fractions from vector-infected, GRK6 (WT)-infected and GRK6 (K215R)-infected NIH3T3 cells. The lysate proteins were labelled with one of the three different fluorescent probes: Vector: Cy2 (shown as blue pseudocolor), GRK6: Cy3 (shown as red pseudocolor) and GRK6 (K215R): Cy5 (shown as green pseudocolor). The labelled proteins in each lysate were mixed together, and the mixture was subjected to two-dimensional difference gel electrophoresis (2D-DIGE) followed by fluorescence scanning ( Fig. 4a ). A small proportion of spots showed a GRK6-induced increase in their acidic forms. We picked out several of these red spots and analysed their protein sequences by mass spectrometry (MS) combined with liquid chromatography. This showed that these proteins were radixin and moesin ( Fig. 4b ), both of which belong to the same protein ezrin/radixin/mosein (ERM) family. These proteins are known to link integral membrane proteins to the cortical actin cytoskeleton located beneath the plasma membrane, thereby contributing to cytoskeletal remodelling [17] and engulfment [29] . Phosphorylation at a carboxy-terminal threonine residue (Thr567 of ezrin, Thr564 of radixin and Thr558 of moesin) has been implicated in the function of ERM family proteins [30] , [31] . Therefore, we first examined whether phosphorylation at these sites was induced by the GRK6 overexpression in NIH3T3 cells. Western blotting using an anti-phosphorylated ERM antibody showed that radixin and moesin phosphorylation was increased in NIH3T3 cells due to GRK6 expression ( Fig. 4c ). This specific phosphorylation was also examined by 2D-western blotting. In this detection system, chemiluminescent signals from the anti-ERM antibody or the phospho-ERM antibody were simultaneously detected with the fluorescent probes used for protein labelling of the lysate mixtures of NIH3T3 cells that expressed WT GRK6 (labelled with Cy3) and GRK6 (K215R) (labelled with Cy5) ( Supplementary Fig. S9 ). Accordingly, we could confirm that these spots had shifted to the more acidic side of the membrane due to GRK6 overexpression and corresponded to phosphorylated ERMs. 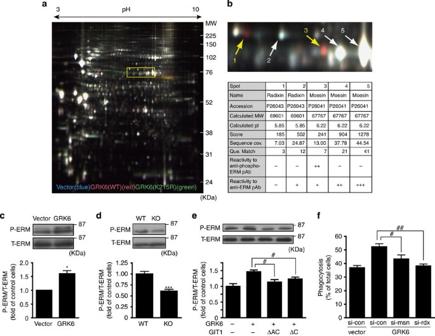Figure 4: Radixin and moesin phosphorylation is induced by GRK6. (a) A representative gel image of 2D-DIGE of phosphoprotein fractions from NIH3T3 cells infected with the empty retrovirus vector (Cy2-labelled, blue), the virus carrying the cDNA for WT GRK6 (Cy3-labelled, red) or GRK6 (K215R) (Cy5-labelled, green). (b) Zoom-in view of an area inarepresenting GRK6 (WT)-induced (yellow arrow, red spot) and unchanged (white arrow, white spot) protein spots. The table summarizes the protein identity, accession number, calculated molecular weight, calculated pI, Mascot score, sequence coverage, query match and reactivity to anti-phospho-ERM antibody that specifically recognizes Thr567 of ezrin, Thr564 of radixin and Thr558 of moesin and anti-ERM antibody for the numbered spots. (c) NIH3T3 cells are retrovirally transfected with GRK6. The cell lysates were subjected to immunoblotting with the anti-phospho-ERM antibody or anti-ERM antibody. Data represent means±s.e.m. (error bars). (d) The cell lysates prepared from BMDMs of WT and GRK6-deficient mice were immunoblotted with the indicated antibodies. Data represent means±s.e.m. (error bars). (e) Cell lysates of NIH3T3 cells infected with the indicated retroviruses were subjected to western blot analysis using anti-phospho-ERM antibody or anti-ERM antibody. (f) GRK6 was transfected with siRNA for control, radixin (rdx) or moesin (msn) and subjected to the engulfment assay. All the experiments were done at least three times, and representative data are shown. *P<0.05, ***P<0.001,#P<0.05 and##P<0.01. KO, knockout; MW, molecular weight; P-ERM, phospho-ERM; T-ERM, total-ERM. Figure 4: Radixin and moesin phosphorylation is induced by GRK6. ( a ) A representative gel image of 2D-DIGE of phosphoprotein fractions from NIH3T3 cells infected with the empty retrovirus vector (Cy2-labelled, blue), the virus carrying the cDNA for WT GRK6 (Cy3-labelled, red) or GRK6 (K215R) (Cy5-labelled, green). ( b ) Zoom-in view of an area in a representing GRK6 (WT)-induced (yellow arrow, red spot) and unchanged (white arrow, white spot) protein spots. The table summarizes the protein identity, accession number, calculated molecular weight, calculated pI, Mascot score, sequence coverage, query match and reactivity to anti-phospho-ERM antibody that specifically recognizes Thr567 of ezrin, Thr564 of radixin and Thr558 of moesin and anti-ERM antibody for the numbered spots. ( c ) NIH3T3 cells are retrovirally transfected with GRK6. The cell lysates were subjected to immunoblotting with the anti-phospho-ERM antibody or anti-ERM antibody. Data represent means±s.e.m. (error bars). ( d ) The cell lysates prepared from BMDMs of WT and GRK6-deficient mice were immunoblotted with the indicated antibodies. Data represent means±s.e.m. (error bars). ( e ) Cell lysates of NIH3T3 cells infected with the indicated retroviruses were subjected to western blot analysis using anti-phospho-ERM antibody or anti-ERM antibody. ( f ) GRK6 was transfected with siRNA for control, radixin (rdx) or moesin (msn) and subjected to the engulfment assay. All the experiments were done at least three times, and representative data are shown. * P <0.05, *** P <0.001, # P <0.05 and ## P <0.01. KO, knockout; MW, molecular weight; P-ERM, phospho-ERM; T-ERM, total-ERM. Full size image We next compared the amounts of the phosphorylated forms of ERMs in BMDMs prepared from WT and GRK6-deficient mice. This revealed that phosphorylated moesin, which is the most abundant and main ERM protein in BMDMs, was significantly decreased in GRK6-deficient BMDMs, which indicated that GRK6 was involved in moesin phosphorylation at its carboxy terminus in vivo ( Fig. 4d ). However, GRK6 did not directly phosphorylate radixin and moesin ( Supplementary Fig. S10 ). ERM phosphorylation by GRK6 was significantly attenuated by the expression of GIT1 mutants that lacked the coiled-coil domain, which suggested that ERM phosphorylation was dependent on the GRK6/GIT1 complex ( Fig. 4e ). In comparison, GRK6-induced ERM phosphorylation was not affected by Y27632, U0126 and LY294002 ( Supplementary Fig. S11 ), which suggested that Rho-kinase, MEK/ERK and phosphatidylinositol-3-kinase were not involved in ERM phosphorylation. When siRNAs for radixin or moesin were transfected into GRK6-overexpressing NIH3T3 cells, engulfment by these cells was markedly attenuated without affecting the GRK6 expression level ( Fig. 4f , Supplementary Fig. S12 ). These results suggest that radixin and moesin phosphorylation contributes to the GRK6-mediated signalling pathway. GRK6-deficient mice exhibit an autoimmune-like disease An in vivo defect in apoptotic cell removal reportedly caused the development of an autoimmune disease that resembled human SLE [32] . Thus, we examined whether GRK6-deficient mice developed autoimmunity. An increase in the amount of anti-dsDNA in serum is one of the most important and reliable criteria for SLE. We first evaluated levels of anti-dsDNA in sera collected from 40-week-old GRK6-deficient and WT mice. Increased anti-dsDNA antibody levels were detected in GRK6-deficient mice ( Fig. 5a ). A major pathogenic consequence of autoantibody production is the deposition of immune complexes in the kidney, which leads to glomerulonephritis. Immunohistochemical analysis of kidney sections showed that there was significantly increased IgG deposition in aged GRK6-deficient mice ( Fig. 5b ). Consistent with IgG deposition, mesangial expansion, which reflects glomerulonephritis, was also observed in the kidneys of GRK6-deficient mice ( Fig. 5c ). In addition, GRK6-deficient mice developed age-dependent splenomegaly that was associated with increased numbers of splenocytes ( Fig. 5d ). At 40 weeks of age, their spleens were approximately 1.6-fold heavier than WT mouse spleens. The white pulp in the spleen was enlarged in GRK6-deficient mice ( Supplementary Fig. S13 ), as was observed in MFG-E8-deficient mice that developed lupus-like autoimmune disease due to the impaired uptake of apoptotic cells [33] . We also examined changes in the lymphoid and myeloid cell populations in the spleens of 40-week-old GRK6-deficient mice. The ratios of B cells to T cells and the frequencies of CD11c + , CD11b + cells and regulatory T cells were similar in WT and GRK6-deficient mice ( Supplementary Fig. S14a–c ). Double staining with anti-CD19 and anti-CD69 antibodies was also similar in GRK6-deficient and WT mice, which indicated that the splenomegaly in GRK6-deficient mice was not due to aberrant B-cell activation ( Supplementary Fig. S14d ). However, the ratio of CD4/CD8 T cells increased in GRK6-deficient mice with a decrease in the CD8 T-cell population, similar to MFG-E8-deficient mice [34] ( Supplementary Fig. S15a ). Therefore, these results support the hypothesis that GRK6-deficient mice developed an autoimmune phenotype, though the symptoms were mild. We also found differences in the CD8 + T-cell populations that mainly affect lupus [34] ( Supplementary Fig. S15b ). Naive T cells (CD44 lo and CD62L hi ) were decreased in GRK6-deficient mice, whereas memory T cells (CD44 hi ) were increased in these mice. CD8 + memory T-cell populations characterized by CD44 expression can be subdivided into effector (low levels of CD62L) and central memory T cells (high levels of CD62L) [35] . In GRK6-deficient mice, the ratio of CD62L lo /CD62L hi cells among the CD8 + memory T-cell population was increased, which indicated that effector memory T cells had increased reminiscent of aged MFG-E8-deficient mice [34] ( Supplementary Fig. S15b ). These results suggested that CD8 + T-cell activation was induced by the increased presentation of apoptotic cell-associated antigens by splenic antigen-presenting cells. In young GRK6-deficient mice at 8 weeks of age, no significant abnormalities were found in their spleen cell subsets ( Supplementary Fig. S16 ). 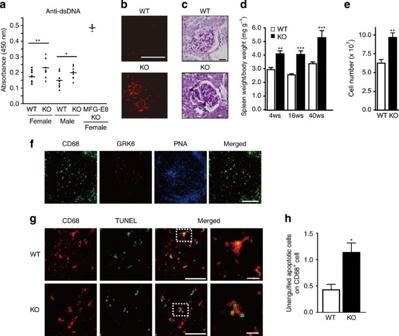Figure 5: GRK6-deficient mice spontaneously develop autoimmune disease. (a) Serum from 40-week-old control WT and GRK6-deficient female (WT:n=14, GRK6-deficient:n=9) and male mice (WT:n=12, GRK6-deficient:n=8) were collected and tested for presence of anti-dsDNA antibodies. Serum from 40-week-old MFG-E8-deficient female mice (n=4) was used as a positive control. (b) Increased deposition of immune complexes in glomeruli of GRK6-deficient mice at 40 weeks of age was assessed by anti-immunoglobulin staining. Scale bar, 100 μm. (c) Paraffin-embedded kidney sections of WT and GRK6-deficient mice at 40 weeks of age were stained using periodic acid-Schiff. Arrowheads indicate a mesangial expansion with increase in matrix and cellularity owing to increased mononuclear cells. Scale bar, 20 μm. (d) Spleens isolated from WT and GRK6-deficient mice of 4-week-old (n=8), 16-week-old (n=4) and 40-week-old (n=9) were weighed, and spleen weight relative to body weight were measured. And the average numbers are shown with s.d. (e) Splenocytes from WT (n=7) and GRK6-deficient mice (n=6) of 40-week-old mice were counted, and the numbers were shown in the graph. (f) Spleen sections from WT mice were stained with anti-CD68 (green), anti-GRK6 (red) and PNA (blue). The fourth column represents the two-colour (anti-CD68 and anti-GRK6) overlay image. Scale bar, 100 μm. (g) Spleen sections from 40-week-old WT and GRK6-deficient mice were double-stained with TUNEL (green) and anti-CD68 antibody (red). Staining profiles were merged in the third column. Scale bar, 50 μm. Enlarged images are shown in the fourth column. Scale bar, 10 μm. (h) The numbers of unengulfed cells associated with CD68-positive macrophages were counted for 40–80 macrophages and are presented as the number per macrophages. The average numbers are shown with s.e.m. All immunohistochemical data are representative of four independent experiments. *P<0.05,**P<0.01 and ***P<0.001. KO, knockout. Figure 5: GRK6-deficient mice spontaneously develop autoimmune disease. ( a ) Serum from 40-week-old control WT and GRK6-deficient female (WT: n =14, GRK6-deficient: n =9) and male mice (WT: n =12, GRK6-deficient: n =8) were collected and tested for presence of anti-dsDNA antibodies. Serum from 40-week-old MFG-E8-deficient female mice ( n =4) was used as a positive control. ( b ) Increased deposition of immune complexes in glomeruli of GRK6-deficient mice at 40 weeks of age was assessed by anti-immunoglobulin staining. Scale bar, 100 μm. ( c ) Paraffin-embedded kidney sections of WT and GRK6-deficient mice at 40 weeks of age were stained using periodic acid-Schiff. Arrowheads indicate a mesangial expansion with increase in matrix and cellularity owing to increased mononuclear cells. Scale bar, 20 μm. ( d ) Spleens isolated from WT and GRK6-deficient mice of 4-week-old ( n =8), 16-week-old ( n =4) and 40-week-old ( n =9) were weighed, and spleen weight relative to body weight were measured. And the average numbers are shown with s.d. ( e ) Splenocytes from WT ( n =7) and GRK6-deficient mice ( n =6) of 40-week-old mice were counted, and the numbers were shown in the graph. ( f ) Spleen sections from WT mice were stained with anti-CD68 (green), anti-GRK6 (red) and PNA (blue). The fourth column represents the two-colour (anti-CD68 and anti-GRK6) overlay image. Scale bar, 100 μm. ( g ) Spleen sections from 40-week-old WT and GRK6-deficient mice were double-stained with TUNEL (green) and anti-CD68 antibody (red). Staining profiles were merged in the third column. Scale bar, 50 μm. Enlarged images are shown in the fourth column. Scale bar, 10 μm. ( h ) The numbers of unengulfed cells associated with CD68-positive macrophages were counted for 40–80 macrophages and are presented as the number per macrophages. The average numbers are shown with s.e.m. All immunohistochemical data are representative of four independent experiments. * P <0.05, ** P <0.01 and *** P <0.001. KO, knockout. Full size image GRK6 is involved in apoptotic cell clearance by macrophages Macrophages in the germinal centre of the spleen are involved in removing apoptotic B cells. Inefficient engulfment by macrophages supposedly triggers immune responses, which results in SLE-like autoimmunity in mice [33] , [36] , [37] . Because we had detected autoimmune properties and abnormalities of the spleen in GRK6-deficient mice, we examined whether GRK6 was expressed by germinal centre macrophages, which were characterized by their CD68 expression. Immunohistochemical staining revealed that GRK6 was expressed in CD68 + macrophages in the germinal centre ( Fig. 5f ). TdT-mediated dUTP nick end labeling (TUNEL)-stained apoptotic cells were also observed in this area ( Fig. 5g ). Furthermore, more TUNEL-positive cells were associated with CD68 + macrophages in GRK6-deficient mice, which indicated that many undigested apoptotic cells were present in the spleens of GRK6-deficient mice ( Fig. 5h ). The numbers of CD68 + macrophages in the white spleen pulp of GRK6-deficient mice were the same as in WT mice, indicating that GRK6 did not affect the development of these macrophages ( Supplementary Fig. S17 ). GRK6 was not involved in the cells’ growth, differentiation or apoptosis ( Supplementary Fig. S18 ). Therefore, GRK6 has an important role in the removal of apoptotic B cells by macrophages in the germinal centre without affecting the development, cell growth, differentiation or apoptosis of these macrophages. We next examined whether the GRK6 expression level was linked to autoimmune diseases. The MRL /lpr mouse is a well-known mouse model of SLE. Immunohistochemical analysis of the spleens from MRL /lpr mice revealed that the GRK6 expression levels in many splenic macrophages of these mice were markedly increased ( Supplementary Fig. S19a,b ), which was accompanied with an increase in the numbers of macrophages ( Supplementary Fig. S19c ). Then, we examined whether GRK6 expression was altered in the macrophages of SLE patients. Among 1,528 autopsies, we could find 6 cases diagnosed with SLE, which is a relatively rare disease. Among these samples, we found an autopsied spleen that had a high expression level of GRK6 in inflammatory cells compared with that of non-SLE patients ( Supplementary Fig. S19d ). GRK6 regulates engulfment of senescent red blood cells Immunohistochemical analysis showed that GRK6 was expressed not only in CD68 + macrophages in the white pulp but also in red pulp macrophages, which was characterized by their expressions of F4/80 + ( Fig. 6a ). Red pulp macrophages have a role in removing senescent red blood cells, thereby contributing to iron recycling in the body. Dead red blood cells express phosphatidylserine, and their clearance is mediated by phosphatidylserine recognition [38] , [39] . Thus, we examined the involvement of GRK6 in the removal of senescent red blood cells, a defect of which leads to iron deposition in the red pulp [40] . Splenic red macrophages isolated from GRK6-deficient mice exhibited a defect in their ability to take up dead red blood cells in vitro ( Fig. 6b ). We also examined the phagocytosis of red blood cells by splenic red pulp macrophages in vivo . Fluorescently labelled dead red blood cells were injected into WT or GRK6-deficient mice. At 24 h after this injection, splenic macrophages were collected and their engulfment capability was analysed. This showed that the engulfment of dead red blood cells by red pulp macrophages was attenuated in GRK6-deficient mice ( Fig. 6c ). Perl’s Prussian staining, which specifically stains iron, revealed that there was increased iron accumulation in the spleen red pulp of GRK6-deficient mice ( Fig. 6d ). Quantitative determinations of the iron contents in spleens also showed that splenic iron concentrations were increased in GRK6-deficient mice ( Fig. 6e ). However, the numbers of red pulp splenic macrophages were not decreased in GRK6-deficient mice ( Fig. 6f ), which indicated that iron deposition was not due to the abnormal development of splenic red pulp macrophages. Expression levels of ferroportin-1, a major iron exporter and hepcidin, an inhibitor of ferroportin-1, were the same in the spleens and livers of WT and GRK6-deficient mice ( Fig. 6g , Supplementary Fig. S20 ). This suggested that iron export was normal in splenic macrophages of GRK6-deficient mice. In addition, GRK6-deficient mice did not exhibit any abnormal red pulp macrophage populations [41] , [42] in their spleens ( Supplementary Fig. S21 ). These results suggested that iron deposition in GRK6-deficient mice was caused by inefficient erythrophagocytosis. However, serum iron parameters and the life spans of red blood cells were normal in GRK6-deficient mice ( Supplementary Tables 1 and 2 and Supplementary Fig. S22 ). 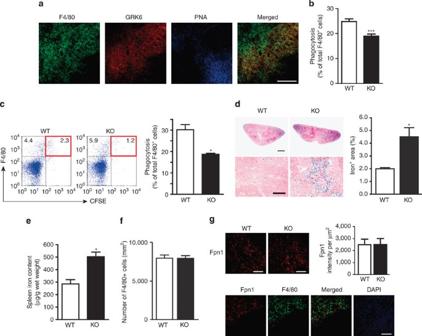Figure 6: GRK6-deficient mice manifest iron accumulation in splenic red pulp. (a) Spleen sections from WT mice were stained with anti-F4/80 antibody (green), anti-GRK6 antibody (red) and peanut agglutinin (PNA) (blue). The fourth column is the merged image of F4/80 and GRK6. Scale bar, 100 μm. (b) Splenic cells from WT and GRK6-deficient mice (1 × 106per well) were co-cultured with CMFDA-labelled apoptotic red blood cells (4 × 107/well) for 90 min at 37 °C. Percentage of F4/80-positive cells carrying the engulfed red blood cells was determined by FACS analysis and shown in the graph. Error bars represent the mean±s.e.m.n=4. (c) Carboxyfluorescein diacetate succinimidyl ester (CFSE)-labelled apoptotic red blood cells were injected to WT and GRK6-deficient mice from tail vein. Percentage of F4/80+splenic macrophage carrying the labelled red blood cells was evaluated by FACS. All numbers within FACS profiles correspond to the percentage of cells within each region. Error bars represent the mean±s.e.m.n=3. (d) Spleen sections from 16-week-old WT and GRK6-deficient mice were stained with Perl’s Prussian blue to visualize the iron deposits. Scale bar, 300 μm. Enlarged images are shown in the lower column. Scale bar, 100 μm. Areas positive for iron staining were quantified and showed as a percentage of the total surface area of the field. The average numbers are shown with s.d.n=3. (e) Iron levels of spleens from 16-week-old WT and GRK6-deficient mice on a standard diet were determined. Error bars represent the mean±s.e.m.n=5. (f) The numbers of F4/80+macrophages in the splenic red pulp were counted in WT and GRK6-deficient mice. The numbers (cells per mm2) were determined by four different fields (0.045 mm2) of spleen sections from WT and GRK6-deficient mice. Error bars represent the mean±s.e.m.n=3. (g) Spleen sections from WT and GRK6-deficient mice were stained with anti-ferroportin-1 (Fpn1) antibody. Fpn1 signal intensity in red pulp areas was determined and showed in the graph. Error bars represent the mean±s.e.m. Representative images of Fpn1 (red) and F4/80 (green), the merged and 4',6-diamidino-2-phenylindole (DAPI) images are shown.n=4. Scale bar, 50 μm. *P<0.05 and ***P<0.001. KO, knockout. Figure 6: GRK6-deficient mice manifest iron accumulation in splenic red pulp. ( a ) Spleen sections from WT mice were stained with anti-F4/80 antibody (green), anti-GRK6 antibody (red) and peanut agglutinin (PNA) (blue). The fourth column is the merged image of F4/80 and GRK6. Scale bar, 100 μm. ( b ) Splenic cells from WT and GRK6-deficient mice (1 × 10 6 per well) were co-cultured with CMFDA-labelled apoptotic red blood cells (4 × 10 7 /well) for 90 min at 37 °C. Percentage of F4/80-positive cells carrying the engulfed red blood cells was determined by FACS analysis and shown in the graph. Error bars represent the mean±s.e.m. n =4. ( c ) Carboxyfluorescein diacetate succinimidyl ester (CFSE)-labelled apoptotic red blood cells were injected to WT and GRK6-deficient mice from tail vein. Percentage of F4/80 + splenic macrophage carrying the labelled red blood cells was evaluated by FACS. All numbers within FACS profiles correspond to the percentage of cells within each region. Error bars represent the mean±s.e.m. n =3. ( d ) Spleen sections from 16-week-old WT and GRK6-deficient mice were stained with Perl’s Prussian blue to visualize the iron deposits. Scale bar, 300 μm. Enlarged images are shown in the lower column. Scale bar, 100 μm. Areas positive for iron staining were quantified and showed as a percentage of the total surface area of the field. The average numbers are shown with s.d. n =3. ( e ) Iron levels of spleens from 16-week-old WT and GRK6-deficient mice on a standard diet were determined. Error bars represent the mean±s.e.m. n =5. ( f ) The numbers of F4/80 + macrophages in the splenic red pulp were counted in WT and GRK6-deficient mice. The numbers (cells per mm 2 ) were determined by four different fields (0.045 mm 2 ) of spleen sections from WT and GRK6-deficient mice. Error bars represent the mean±s.e.m. n =3. ( g ) Spleen sections from WT and GRK6-deficient mice were stained with anti-ferroportin-1 (Fpn1) antibody. Fpn1 signal intensity in red pulp areas was determined and showed in the graph. Error bars represent the mean±s.e.m. Representative images of Fpn1 (red) and F4/80 (green), the merged and 4',6-diamidino-2-phenylindole (DAPI) images are shown. n =4. Scale bar, 50 μm. * P <0.05 and *** P <0.001. KO, knockout. Full size image We finally compared iron deposition in the spleens of GRK6-deficient mice with that in WT mice after acute anaemia. Acute haemolysis induced by injecting phenylhydrazine is accompanied by shrinkage of the white pulp and causes an enlargement of the red pulp due to an influx of dead red blood cells [43] ( Supplementary Fig. S23a ). More iron was deposited in the spleens of GRK6-deficient mice after phenylhydrazine injection ( Supplementary Fig. S23b ). Similar results were obtained after inducing acute anaemia by phlebotomy ( Supplementary Fig. S23c ). GRK6 is a member of the GRK family of proteins that were initially identified as kinases responsible for the desensitization and downregulation of GPCRs. In this report, we identified GRK6 as an important molecule that promotes efficient apoptotic cell engulfment by several types of macrophages. A deficiency of this molecule resulted in an autoimmune-like disease and splenic iron accumulation in these mice. GRK6-mediated engulfment was largely independent of two well-established intracellular engulfment pathways, DOCK180/ELMO/Rac1 and GULP/Rac1, but did require GIT1 and the phosphorylation of radixin and moesin. Both GRK2 and GRK6 expressions enhanced apoptotic engulfment. However, the promotion of apoptotic cell engulfment by GRK6 but not GRK2 depends on its kinase activity. A previous report showed that GRK2 positively regulated integrin-dependent epithelial cell migration in a kinase activity-independent manner, which was orchestrated by GIT1 [20] . The function of GRK2 in cell migration was regulated by its phosphorylation at certain tyrosine and serine residues [20] , [44] , which led to the interaction of GRK2 with GIT1. This interaction modulates the Rac1/PAK/MEK/ERK1/2 pathway in response to sphingosine-1-phosphate and adhesion [20] . In contrast, the GRK6–GIT1 complex did not significantly influence this pathway ( Supplementary Fig. S8 ). Considering these differences, the pro-migratory or pro-engulfmental signal transduction pathway mediated by GRK2 [44] , [45] or GRK6 is regulated by distinct molecular mechanisms, although GIT1 is common to both the pathways. GRK2 was reported to directly phosphorylate ERM [46] , whereas it did not undergo direct phosphorylation by GRK6. This may also contribute to the different signalling pathways by the two GRKs. The molecular mechanism by which GRK2 or GRK6 defines its specific signal transduction pathway will be an interesting theme for future studies. With regard to the clearance of senescent red blood cells by splenic macrophages, the CD47-SHPS-1 regulatory system has been well studied [47] . The CD47-SHPS-1 system defines self- and non-self recognition by macrophages, which generates the so-called ‘Don’t eat me signal’ that enables viable red blood cells to escape engulfment by phagocytes. In this study, we found that GRK6 promoted the engulfment of senescent red blood cells by red splenic macrophages and contributed to iron homoeostasis. A recent report [40] showed that Spic-deficient mice selectively lost splenic red pulp macrophages. In these mice, iron deposition in their spleens was observed due to the inefficient engulfment of dead red blood cells. In spite of this iron deposition, Spic-deficient mice did not show any significant abnormalities in total iron homoeostasis, which was similar to GRK6-deficient mice. To date, studies on the diseases of iron metabolism have usually focused on the proteins that directly alter iron transport, such as iron transporters/exporters, receptors for iron-binding proteins or the regulators of the activities of these transporters and receptors. Our study provides a new model of human iron disorders in the spleen. GRK6 may be a candidate gene that is responsible for iron overload in some patients. In summary, we revealed that GRK6 was involved in apoptotic cell clearance by two independent subsets of macrophages in the spleen. GRK6 greatly contributed to removing unnecessary B cells by splenic white pulp macrophages and removing senescent red blood cells by splenic red pulp macrophages. However, we cannot rule out the possibility that some unidentified roles for GRK6, other than engulfment, influence the phenotypes of GRK6-deficient mice, as our experiments were performed using GRK6 systemic knockout mice. Thus, to conclude that the phenotypes observed here were due to engulfment defects by GRK6-deficient macrophages, it will be necessary to examine the phenotypes of GRK6-deficient mice after transplanting bone marrow cells from WT mice and vice versa. In vitro phagocytosis assay For uptake assays in vitro , we used apoptotic thymocytes or red blood cells as preys. Thymocytes or red blood cells from 4- to 8-week-old C57BL/6 mice were isolated and labelled with 1 μM CMFDA (Life Technologies) by incubating them at 37 °C for 30 min. After the labelling, the thymocytes were allowed to undergo apoptosis by treating thymocytes with 10 μM dexamethasone for 4 h at 37 °C. The labelled red blood cells were suspended in PBS and incubated in the incubator (5% CO 2 , 37 °C) for 24 h to induce apoptosis. The labelled apoptotic thymocytes or apoptotic red blood cells were added on the NIH3T3 cells (4 × 10 4 cells) and BMDM (2 × 10 5 cells) or splenic macrophages (1 × 10 6 cells), respectively, in a 24-well plate and co-cultured at 37 °C. The NIH3T3 cells, BMDM and splenic macrophages were vigorously washed by PBS, followed by the treatment with 0.2% trypsin containing 1 mM EDTA. The detached cells were analysed by flow cytometry using a FACS Calibur (BD Biosciences). GTP-Rac1 pull-down assay Retrovirus-infected cells were lysed by GTP-Rac1 pull-down assay buffer (50 mM Tris-Cl (pH 7.5), 0.1% Triton X-100, 10% glycerol, 150 mM NaCl, 30 mM MgCl 2 , 1 mM DTT, 1 mM PMSF, 2 μg ml −1 leupeptin and 10 μM pepstatin). The lysates were collected and centrifuged at 15,000 r.p.m. for 10 min at 4 °C to remove cell debris. An amount of 10 μg GST-PAK-Rac1/Cdc42 binding domain and 30 μl Glutathione-Sepharose beads were added to each lysate. The mixtures were incubated at 4 °C for 1 h with gentle rotation. After the incubation, they were subjected to a wash by using the pull-down assay buffer and a brief centrifuge (5,000 r.p.m. for 1 min). The wash was repeated twice and, finally, the beads were boiled in 60 μl SDS sample buffer for 5 min at 95 °C. After the centrifuge, the samples were analysed by western blotting using anti-Rac1 antibody (BD Transduction). In vivo phagocytosis assay For splenic macrophage uptake assays, we intravenously injected 8 × 10 7 CMFDA-labelled apoptotic thymocytes into 10- to 12-week-old WT or GRK6-deficient mice. Two hours after the injection, the mice were killed and their spleens were extirpated. The spleens were smashed between two glass slides, and single-cell splenocyte suspensions were stained with anti-CD11b-APC to identify macrophage population after lysis of red blood cells. Cells were analysed by flow cytometry. Engulfment of red blood cells in vivo Red blood cells isolated from WT mice were suspended in 30 ml PBS and incubated with 5 μM carboxyfluorescein diacetate succinimidyl ester (Invitrogen) for 10 min at room temperature. After the incubation, the cells were washed three times by PBS and suspended in 2 ml PBS. The cell suspension of 200 μl was injected into WT or GRK6-deficient mice. Twenty-four hours after the injection, spleens of the mice were isolated and minced. The isolated splenocytes were stained with anti-F4/80-APC and analysed by flow cytometry. Immunoprecipitation NIH3T3 cells or transfected HEK293 cells expressing Flag-GRK6 and HA-GIT1 were washed and scraped by lysis buffer 1 (50 mM HEPES (pH 7.5), 250 mM NaCl, 2 mM EDTA, 10% glycerol, 0.5% NP40, 1 mM Na 3 VO 4 and 1 mM NaF) containing protease inhibitors (Nacalai). The scraped cells were incubated on ice for 30 min and centrifuged at 14,000 r.p.m. for 10 min at 4 °C. The supernatant was collected and rotated gently for 90 min at 4 °C after adding 20 μl anti-Flag antibody beads (Sigma). In the experiment to detect the endogenous interaction between GRK6 and GIT1 in BMDM, the cells were lysed in lysis buffer 2 (50 mM Tris-Cl (pH 7.5), 300 mM NaCl, 0.1% SDS, 1% Triton X-100, 0.5% Sodium deoxycholate, 1 mM Na 3 VO 4 and 1 mM NaF) containing protease inhibitors (Nacalai). The lysed cells were incubated on ice for 15 min and centrifuged at 14,000 r.p.m. for 10 min at 4 °C. The collected supernatant was then incubated with anti-GRK6 antibody (Santa Cruz Biotechnology) overnight at 4 °C, followed by the incubation with Protein A-Sepharose beads (GE Healthcare) for 2 h. After the incubation, the beads were washed three times by lysis buffer 1 or 2 of 1,000 μl, and 20 μl SDS sample buffer was added to the beads and they were boiled for 5 min at 95 °C. After centrifugation, the supernatant was collected and subjected to SDS gel electrophoresis and western blotting with antibodies (mouse anti-HA (1:2,000 dilution; Roche), rabbit anti-GIT1 (1:2,000 dilution; Santa Cruz Biotechnology), rabbit anti-GRK6 (1:4,000 dilution; Santa Cruz Biotechnology) and horseradish peroxidase-conjugated anti-mouse IgG (1:5,000 dilution; Santa Cruz Biotechnology) or anti-rabbit IgG (1:5,000 dilution; Santa Cruz Biotechnology). Two-dimensional difference gel electrophoresis Phosphoprotein-enriched fractions were subjected to 2D-DIGE essentially as described previously [28] . Briefly, total cell lysates were prepared from NIH3T3 cells overexpressing vector alone, GRK6 or GRK6 (K215R). Then, phosphoproteins in each cell lysate were enriched by using the Phosphoprotein Purification Kit (Qiagen), and interfering nonprotein material was subsequently removed (2-D Clean-Up Kit; GE Healthcare). Thirty microgram of the resultant phosphoprotein-enriched fractions were minimally labelled with 400 pmol Cy2, Cy3 or Cy5 fluorescent dye (CyDye DIGE Fluors, GE Healthcare) for 30 min on ice. After quenching the labelling reaction with 10 nmol lysine, these differentially labelled samples were mixed and subjected to first-dimension isoelectric focusing on immobilized pH gradient strips (24 cm; pH 3–10 non-linear) using an Ettan IPGphor II system. The second-dimensional SDS–PAGE was carried out on 9% acrylamide gel. The Cy2, Cy3 and Cy5 signals were individually acquired with a Typhoon 9400 scanner (GE Healthcare). Protein identification by MS After obtaining fluorescent images, the 2D-DIGE gel was silver-stained (Thermo Fisher Scientific/Pierce). Protein spots were excised and digested with trypsin (Promega). The resultant peptides were analysed by a capillary liquid chromatography system (Waters/Micromass, Manchester, UK) connected to a Q-TOF2 mass spectrometer (Waters/Micromass). Raw data were acquired and processed using MassLynx version 4.0. (Waters/Micromass) to generate a peak list file for MS/MS ion search. The peak list files were searched against the NCBI non-redundant protein database restricted to Mus musculus using the MS/MS ion search on Mascot search engine (Matrix Science). Immunohistochemistry Cryosections (4 μm) of the spleen of WT or GRK6-deficient mice were fixed in cold acetone for 10 min and blocked with PBS containing 3% BSA for 1 h. After the blocking, the slides were incubated with anti-GRK6 (1:50 dilution; Santa Cruz Biotechnology), anti-CD68 (1:200 dilution; Serotec), anti-F4/80 (1:200 dilution; Serotec) and PNA (1:50 dilution; Vectashield) overnight at 4 °C, followed by staining with fluorescent-conjugated secondary antibodies. For staining with an antibody against ferroportin-1, livers and spleens of mice were fixed with 4% paraformaldehyde (PFA) overnight at 4 °C and embedded in FSC22 Frozen Section Media (Leica Microsystems). Tissue sections (6 μm in thickness) were blocked with 3% BSA and reacted with anti-ferroportin-1 (1:200; Alpha Diagnostics) overnight at 4 °C. Then, the sections were incubated with AlexaFluor 594 goat anti-rabbit antibody (Invitrogen). TUNEL assays were performed according to the manufacturer’s instructions (ApopTag Fluorescein Direct In Situ Apoptosis Detection Kit; Millipore). For detection of immune complex in the kidney, 40-week-old mouse kidneys were fixed with 4% PFA and embedded in OCT compound (Tissue-Tek). Kidney sections that were 4-μm thick were blocked with PBS containing 3% BSA and stained with Cy3-conjugated F(ab′)2 of goat anti-mouse IgG (Jackson ImmunoResearch Laboratories). Perl’s Prussian blue stain or hematoxylin and eosin stain was performed according to the manufacturer’s protocol (Sigma) by using paraffin-embedded spleen sections fixed by 4% PFA. Kidney sections fixed with 4% PFA were subjected to periodic acid-Schiff stain according to the standard procedures. All the stained sections were observed under a fluorescence microscope (Keyence BZ-9000) or a confocal microscope (Olympus FV10i or Nikon A1Rsi). Enzyme-linked immunosorbent assay The serum from 40-week-old WT, GRK6-deficient and MFG-E8-deficient mice was diluted 25 times in PBS, and 100 μl of the diluted serum was added on the 96-well enzyme-linked immunosorbent assay plates coated with double-stranded DNA (Mesacup DNA-II test; MBL). One hour after the incubation at room temperature, the serum was removed and the plates were incubated with horseradish peroxidase-conjugated goat antibody against anti-mouse Ig (G+M+A) (Cappel) for 1 h. The peroxidase activity was detected by the Peroxidase Detection Kit (Sumitomo), and the absorbance of 450 nm was measured by a microplate reader (Berthold Technologies). Measurement of iron concentration in spleen Spleens were weighed and digested in 10% trichloroacetic acid with homogenizer and incubated at 65 °C for 24 h with agitation. The solution was centrifuged at 14,000 r.p.m. for 5 min. The supernatant was collected and neutralized with NaOH to adjust pH >2. The resultant solution was subjected to iron measurement by Mettaloassay LS-MPR Kit (AKJ Global Technology, Japan) based on Nitroso-PSAP method according to the manufacturer’s protocol. The absorbance of 750 nm was determined by using a spectrometer. Statistical analysis The results are represented as means±s.e.m. from at least three independent experiments. We employed Student’s t -test for comparisons for two groups and analysis of variance with the Student–Newman–Keuls test for multiple-group comparison. How to cite this article: Nakaya, M. et al . GRK6 deficiency in mice causes autoimmune disease due to impaired apoptotic cell clearance. Nat. Commun. 4:1532 doi: 10.1038/ncomms2540 (2013).